Graphene-enabled electrically switchable radar-absorbing surfaces Radar-absorbing materials are used in stealth technologies for concealment of an object from radar detection. Resistive and/or magnetic composite materials are used to reduce the backscattered microwave signals. Inability to control electrical properties of these materials, however, hinders the realization of active camouflage systems. Here, using large-area graphene electrodes, we demonstrate active surfaces that enable electrical control of reflection, transmission and absorption of microwaves. Instead of tuning bulk material property, our strategy relies on electrostatic tuning of the charge density on an atomically thin electrode, which operates as a tunable metal in microwave frequencies. Notably, we report large-area adaptive radar-absorbing surfaces with tunable reflection suppression ratio up to 50 dB with operation voltages <5 V. Using the developed surfaces, we demonstrate various device architectures including pixelated and curved surfaces. Our results provide a significant step in realization of active camouflage systems in microwave frequencies. Microwaves are part of the electromagnetic spectrum with wavelengths of from one millimetre to a metre. Radar and communication technologies use passive metallic surfaces to guide microwaves in the free space and resistive surfaces to absorb them [1] , [2] . Although the source of microwaves can be controlled by electrical means, active control of microwaves in the free space has been a challenge due to the requirement of large-area adaptive surfaces in microwave frequencies [3] , [4] , [5] , [6] , [7] , [8] . Microwave analogues of smart optical windows that enable electrically tunable microwave reflection and transmission have been the subject of active research for many decades [3] , [7] , [9] . The key challenge is the ability to tune the interaction between microwaves and matter by electrical means. These interactions are mainly governed by dielectric response of the materials. Materials with tunable conductivity [9] , [10] , permittivity [11] or permeability [12] , [13] have been exploited for adaptive surfaces. Instead of controlling the bulk material properties, here we propose to control microwaves by tuning the density of free charges on a surface. Large-area, the two-dimensional crystal of carbon, graphene, allows us to test this approach and fabricate a new class of adaptive microwave surfaces [14] , [15] . One can confidently argue that an atomically thin coating has negligible effects on the reflection of microwaves from a surface unless there are abundant free charges on it. Through electrostatic doping, we show that atomically thin layers can be used as a switchable radar absorbing surfaces. Graphene and carbon nanotube-based composite materials have been used as resistive materials to absorb microwaves; however, to our knowledge they have not been used for active microwave surfaces [16] , [17] , [18] , [19] , [20] , [21] , [22] , [23] , [24] , [25] , [26] , [27] . Metals do not yield tunable electrical conductivity via external electric fields. This drawback prevents the uses of metals for adaptive microwave surfaces. Semiconductors can yield tunable surface charge density by means of metal-oxide semiconductor structures [28] ; however, the metallic gate electrode covers the surface of semiconductor and screens the accumulated charges. Heating or illuminating a bare semiconductor surface with a light source can generate free carriers; but, these techniques are not practical for realistic device configurations. Electrically tunable materials such as ferroelectric materials [29] , [30] and composite polymers [31] , [32] have been studied for possible active microwave surfaces. Inability to fabricate these materials over large area and weak modulation of dielectric properties prevents realization of adaptive microwave surfaces. Another approach is to use distributed active circuit elements (diodes, transistors or photo-switches) integrated with passive metallic structures [33] , [34] . External bias voltage or light source applied on these distributed circuit elements changes the effective length of metallic structures, which yield limited control over the reflectivity of the surface. Moreover, micro-electro-mechanical devices and mechanical actuators have been used to control microwaves by mechanical means [35] , [36] . Recently, graphene provides new perspective to realize adaptive surfaces. The ability to control charge density on graphene enables new active terahertz devices for various applications such as switches [37] , modulators [38] , [39] , [40] , [41] , [42] , metamaterials [43] , [44] , [45] , plasmonics [44] , [46] and cloaking [43] , [47] . A review by Sensale–Rodrigues et al. [48] summarizes these recent developments in reconfigurable terahertz optoelectronics. The physical mechanism of these active THz devices is based on controlling intraband transitions of graphene. In this paper, we implement the same idea to microwave frequencies to realize switchable radar-absorbing surfaces. Owing to the centimetre scale wavelength, adaptive microwave surfaces require challenging growth and device considerations. We show that large-area graphene capacitors eliminate these challenges and provide electrically reconfigurable surfaces, which would function as electrically switchable radar-absorbing surfaces. Monoatomic thickness, tunable high mobility charged carriers together with the large-area synthesis of graphene provide unique configuration for the realization of the adaptive microwave surfaces. 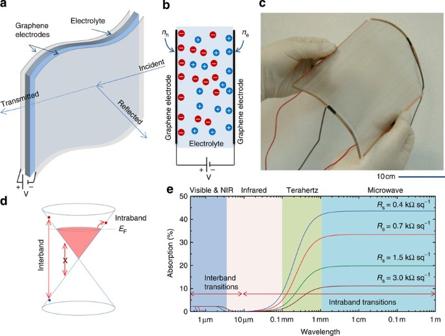Figure 1: Graphene capacitors as broadband adaptive surfaces. (a) Schematic representation of the graphene-based adaptive microwave surfaces. The device consists of two large-area graphene electrodes transfer printed on a microwave-transparent PVC support and electrolyte between them. (b) Cross-sectional view of the device. Application of a voltage bias polarizes the electrolyte (ionic liquid) and forms ionic double layers on the graphene–electrolyte interface. (c) Photograph of the fabricated device. (d) Representation of the electronic band structure of graphene and electronic transitions that define the broadband optical response. (e) Calculated broadband absorption of a single-layer graphene with different sheet resistance for the electromagnetic spectrum covering from the visible to microwave frequencies. Adaptive microwave surfaces Figure 1a shows a schematic representation of the device that functions as an adaptive microwave surface. The working principle of the device is based on the electrostatic tuning of high mobility carriers on graphene electrodes without using metallic structures. The device consists of two large-area graphene electrodes on flexible polymer support and electrolyte medium between them. The cross-sectional view of the device is shown in Fig. 1b . Application of a bias voltage between the graphene electrodes polarizes the electrolyte and forms ionic double layers on the graphene–electrolyte interface with opposite polarizations. These ionic double layers generate tunable high-mobility free carriers (electrons and holes) on the graphene electrodes that can respond to microwaves. Reflection due to the electrolyte is negligible, because the ions of the electrolyte have very low mobility; therefore they cannot respond to the electric field of microwaves ( Supplementary Table 1 ). To fabricate this device, we synthesized large-area graphene (20 cm × 20 cm) by chemical vapour deposition on ultra-smooth copper foils and then transferred it on a microwave-transparent and flexible polyvinyl chloride substrate (PVC, thickness of 70 μm, see Supplementary Fig. 1 ). We attached two graphene-coated PVC films (graphene-coated sides are facing to each other and separated by 50-μm thick spacer) and filled the gap between graphene electrodes with ionic liquid (diethylmethyl(2-methoxyethyl)ammonium bis(trifluoromethylsulfonyl)imide, [deme][Tf2N]), which works as an electrolyte with a wide electrochemical window of ±3.5 V. Figure 1c shows the fabricated device with dimensions of 20 cm × 20 cm. This simple device architecture yields an unprecedented ability to control charge density on large-area graphene electrode, which operates as a tunable metal. Electrostatic and electrochemical mechanisms are used to store charges at the electrode of the supercapacitors. In our devices, we used only electrostatic storage to prevent detrimental effects on single-layer graphene. Redox reactions can damage the electrical continuity of the single-layer graphene. Electrochemical storage can be used for multilayer graphene electrodes; however, multilayer graphene is not suitable for our purpose due to the lack of efficient modulation. Figure 1: Graphene capacitors as broadband adaptive surfaces. ( a ) Schematic representation of the graphene-based adaptive microwave surfaces. The device consists of two large-area graphene electrodes transfer printed on a microwave-transparent PVC support and electrolyte between them. ( b ) Cross-sectional view of the device. Application of a voltage bias polarizes the electrolyte (ionic liquid) and forms ionic double layers on the graphene–electrolyte interface. ( c ) Photograph of the fabricated device. ( d ) Representation of the electronic band structure of graphene and electronic transitions that define the broadband optical response. ( e ) Calculated broadband absorption of a single-layer graphene with different sheet resistance for the electromagnetic spectrum covering from the visible to microwave frequencies. Full size image Notably, tunable charge density on large-scale graphene enables us to control light–matter interaction in a very broad spectrum ranging from the visible to microwave frequencies [42] , [48] , [49] , [50] , [51] . Figure 1d illustrates the interband and intraband electronic transitions of graphene that define this broadband optical response. We calculated the optical absorption of single-layer graphene with different charge densities over a very broad spectrum covering from the visible to microwave ( Fig. 1e ). We can classify this spectrum into two sections based on interband and intraband transitions. The optical response in the visible and near-infrared is defined by the interband transitions, which provide a constant optical conductivity, and yield 2.3% broadband optical absorption and negligible reflection. This small absorption can be blocked via Pauli blocking that yields step-like optical transmission spectra with a cutoff at 2 E F . To obtain the charge density on graphene electrodes, we measured the Fermi energy from the optical transmission spectra (500–1,100 nm range, Supplementary Figs 2 and 3 ). Fermi energy of graphene electrodes scales with the charge density as where v F is the Fermi velocity (1.1 × 10 8 cm s −1 ) [52] and n is the charge density. As ionic liquid electrolyte yields very efficient electrostatic doping, the Fermi energies increase up to 1 eV ( Supplementary Fig. 2 ) at a bias voltage of 5 V. The extracted charge density on graphene electrodes varies between 0.5 × 10 13 to 5.5 × 10 13 cm −2 . The associated Fermi energies vary between 0.2 and 1 eV. For longer wavelengths, however, interband transitions are blocked due to unintentional doping; therefore, the long-wavelength optical response is due to intraband transitions, which yield frequency-dependent Drude-like optical conductivity [50] of σ ( ω )= σ DC /(1− iωτ ), where σ DC is the low-frequency conductivity, ω is the angular frequency of electromagnetic wave and τ is the electron scattering time. By tuning the low-frequency conductivity of graphene through electrostatic doping, we can obtain significant change in the absorption (as large as 50%) in the microwave frequency. This large broadband absorption has been predicted for ultrathin conducting films [53] and graphene [42] . The absorption due to intraband transitions rolls down at terahertz frequencies ( ) due to the electron scattering time of graphene. The electron relaxation time for CVD graphene is around 0.2 ps (ref. 54 ), which corresponds a cutoff frequency of 5 THz. Therefore, we expect that the response of graphene supercapacitors to be flat in the microwave frequencies and rolls down in the THz frequencies [38] , [42] . We measured the microwave reflection and transmission from our device at a frequency of 10.5 GHz (wavelength of 2.8 cm). We used a TE-polarized microwave transmitter with a power of 15 mW and two receivers ( Fig. 2a ). We applied an external voltage bias and measured the variation of the reflected ( Fig. 2b ) and transmitted ( Fig. 2c ) microwave power. At a bias voltage of 0 V, only 1.8% of the incident beam is reflected from the device. This small reflection is due to the residual charges and/or unintentional doping on the graphene electrodes. The PVC substrate and the ionic liquid have negligible microwave reflection (<0.1%, Supplementary Table 1 ). As we increase the bias voltage, the reflection increases up to 20% at a bias voltage of 3.5 V. As the charge density on the capacitor increases, the transmitted power decreases from 76 to 36% because of enhanced reflection and absorption. The extracted microwave absorption due to Joule heating ( A= 1 −T−R where T and R refer transmitted and reflected power) is given in Fig. 2d . The microwave absorption of the graphene capacitor can be tuned between 21 and 45% of the incoming microwaves for the bias voltage range of 0–3.5 V. We observed a slight asymmetry in modulation of microwaves at positive and negative voltages likely due to different ionic strength of anions and cations of the electrolyte. The sheet resistance of the graphene electrodes is a practical parameter to understand the microwave response of this device. 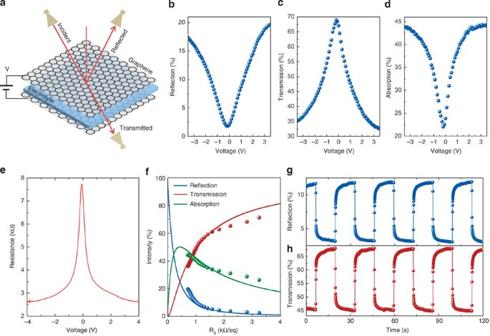Figure 2: Microwave characterization of the adaptive microwave surfaces. (a) Experimental set-up used for the microwave measurements. A microwave transmitter with a power of 15 mW at 10.5 GHz and two receivers were used to measure the reflected and transmitted microwave power. (b,c) Measured intensity of the reflected and transmitted microwaves plotted against the bias voltage. (d) The extracted microwave absorption of the graphene capacitor as a function of bias voltage. (e) Measured resistance of graphene electrodes (including contact resistance) as a function of bias voltage. (f) The experimental (scattered plot) and calculated (solid lines) microwave reflection, transmission and absorption are plotted against sheet resistance. (g,h) Real-time microwave reflection, and transmission, through the graphene capacitor during periodic charging and discharging. The RC response time of the capacitor is determined by the varying resistance of the graphene electrodes and the total capacitance of the device. The extracted response time of graphene capacitor with dimensions of 8 × 8 cm2is around 300 ms. Figure 2e shows the variation of the total resistance of the device as a function of bias voltage. The total resistance ( R T +R B , T and B represents the top and bottom electrodes) reaches the peak value of 8 kω at the charge neutral point (−0.1 V) and decreases down to 2.7 kΩ at a bias voltage of 3.5 V. After extracting the contact resistance ( R c ~0.8 kΩ, Supplementary Fig. 4 ), we plot the measured values of the reflection, transmission and absorption of microwaves at 10.5 GHz frequency, against the sheet resistance of the graphene electrode ( Fig. 2f ). We also observed small hysteresis when we switched the scan direction ( Supplementary Figs 5 and 6 ). There are two mechanisms that cause the observed hysteresis in our devices. The first mechanism is the formation of electrical double layers and slow response of the electrolyte due to low mobility of the ions in the electrolyte. Hysteresis during charging and discharging is a common phenomenon in supercapacitors. The second mechanism is the electrochemical doping of graphene electrodes. When we apply relatively large voltage, which is close to the electrochemical window, the small leakage current ( Supplementary Fig. 7 ) induces chemical doping on graphene, which shifts the Dirac point. The shift in Dirac point during the voltage scan appears as a hysteresis in the microwave measurements. To get more insight, we calculated the coefficient of reflection and transmission of graphene electrodes for TE-polarized electromagnetic waves by solving the Maxwell’s equations for the capacitor geometry (two graphene electrodes and ionic liquid between them, see Supplementary Note 1 ). We modelled graphene as a Drude metal with a frequency dependent conductivity σ ( ω )= σ DC /(1− iωτ ), where σ DC is the low-frequency conductivity, ω is the angular frequency of electromagnetic wave and τ is the electron scattering time (150 fs) [55] . At 10.5 GHz, the conductivity is very close to σ DC obtained from the transport measurements. The results of the electromagnetic model is plotted in Fig. 2f (line plot) against the sheet resistance of the graphene layers. As the sheet resistance of graphene increases, the microwave reflection drops sharply, whereas the microwave transmission increases. Interestingly, the microwave absorption reaches a maximum of 50% at the sheet resistance of 430 Ω and drops gradually as the sheet resistance increases further. We observed a good agreement between the experiment and the electromagnetic model. The slight deviation at large sheet resistance (around Dirac point) is likely because of inhomogeneous charge density on large-area graphene owing to the charge puddle formation [56] . The variation of the microwave reflection can be understood by a simple transmission line model ( Supplementary Note 2 ). As the sheet resistance of graphene varies, the characteristic impedance of the surface changes. The dynamic range of the microwave surface is limited by the two main effects: (1) the electrochemical window of the electrolyte, which limits the maximum charge density on graphene electrodes, (2) the unintentional doping on the graphene, which limits minimum charge density. However, due to the lack of a band gap, there is always some degree of charges on graphene electrodes at unbiased case. A graphene-like material with electronic band gap (carbon nanotube networks, MoS 2 or other 2D materials) could provide better control of the minimum charge density. Thermal effects due to the absorbed microwaves on graphene electrodes is another limiting factor for high microwave powers. The thermal effects can be optimized by controlling the substrate material and the geometry. Figure 2: Microwave characterization of the adaptive microwave surfaces. ( a ) Experimental set-up used for the microwave measurements. A microwave transmitter with a power of 15 mW at 10.5 GHz and two receivers were used to measure the reflected and transmitted microwave power. ( b , c ) Measured intensity of the reflected and transmitted microwaves plotted against the bias voltage. ( d ) The extracted microwave absorption of the graphene capacitor as a function of bias voltage. ( e ) Measured resistance of graphene electrodes (including contact resistance) as a function of bias voltage. ( f ) The experimental (scattered plot) and calculated (solid lines) microwave reflection, transmission and absorption are plotted against sheet resistance. ( g , h ) Real-time microwave reflection, and transmission, through the graphene capacitor during periodic charging and discharging. The RC response time of the capacitor is determined by the varying resistance of the graphene electrodes and the total capacitance of the device. The extracted response time of graphene capacitor with dimensions of 8 × 8 cm 2 is around 300 ms. Full size image To probe the switching characteristics of the active microwave surface, we monitored the reflected and transmitted microwave power as the bias voltage varies repeatedly between 3 and 0 V. Figure 2g,h shows the time trace of the reflected and transmitted power, respectively. The graphene capacitor behaves like a nonlinear RC circuit ( Supplementary Figs 12–14 ). The response time of the device is characterized by the resistance of graphene electrodes and the capacitance of the device. We extracted the response time of 300 ms for a device with dimensions of 8 × 8 cm 2 . This number agrees well with averaged time constant τ=RC =330 ms calculated from the average capacitance (~100 μF) and resistance (~3.3 kΩ sq −1 ) obtained from the transport measurements. The time constant of the device can be reduced by increasing the charge mobility of graphene electrodes (that is, increasing the grain size of graphene flakes) or ionic mobility of the electrolyte. Using an electrolyte with high ionic conductivity can improve the response time; however, there is a trade of between the ionic mobility and electrochemical stability. The ionic liquid electrolyte [deme][Tf2N] provides the optimum performance (see Supplementary Table 1 ) [57] . Switchable radar-absorbing surfaces After studying the microwave response of the graphene capacitors, we would like to demonstrate electrically switchable radar-absorbing surfaces. The maximum microwave absorption of single-layer graphene is limited to 50% defined by the Maxwell’s equations [42] , [53] . To reduce the microwave reflection from the surface, we demonstrated a resonant device architecture ( Fig. 3a ) that includes the graphene capacitor and a flat metallic surface, placed at a distance of quarter of the wavelength ( , where, λ is the wavelength and θ is the incidence angle). This configuration is known as Salisbury screen previously used for enhancing microwave absorption of resistive materials [5] and graphene at infrared and terahertz frequencies [38] , [58] . 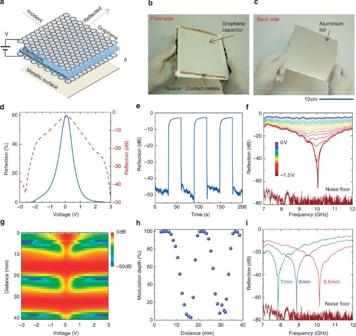Figure 3: Graphene-based switchable radar-absorbing surfaces. (a) Schematic representation of the resonant device including the graphene capacitor and metallic surface placed at a distance of quarter-wavelength. (b,c) Photographs of the front and the back side of the fabricated device. (d) The measured microwave reflection at 10.5 GHz plotted against the bias voltage. The red curve shows the reflection in decibel. (e) Real-time reflection from the device during periodic charging and discharging. The device yields around 50 dB reflection suppression ratio. (f) Broadband reflection spectrum from the device at various bias voltages. The noise floor is at −80 dB. (g) Microwave reflection from the device plotted against the bias voltage and the spacer thickness, which defines the distance between the graphene electrodes and metallic surface. (h) Variation of the modulation depth of the resonant device with the spacer thickness. When the graphene is at the antinodes, the modulation is around 100%, whereas at the nodes the modulation is close to zero. (i) Broadband reflection spectra from the device for three different spacer thickness. Figure 3b,c shows the pictures of the front and back side of the resonant device. Surprisingly, placing a flat metal at a suitable distance yields very high reflection suppression at high doping concentration on graphene. The variation of the microwave reflection of this device is shown in Fig. 3d . At 0 V, the reflection is maximum at 60% (−3 dB) and as we increase the bias voltage, the reflection diminishes entirely (<−45 dB, Fig. 3d ). At 3 V, the Fermi energy and charge density on graphene electrodes are around 0.95 eV and 5.5 × 10 13 cm 2 , respectively. The time traces of the reflection ( Fig. 3e ) shows a remarkable reflection suppression ratio of around 50 dB, which is limited by our detector. When the gap between the graphene electrodes and the metallic surface is a quarter of the wavelength, the reflection from the metallic surface forms a standing wave with the antinodal plane (maximum lateral electric field), which is on graphene electrode. Therefore, the distance between the graphene electrodes and the metallic surface defines the modulation depth ( , R on and R off represent the reflected power at the on- and off-state). Figure 3h shows the variation of the modulation depth with the distance. Interestingly, when the distance is half-wavelength (graphene electrodes are at the nodes of the standing wave), we do not observe any modulation in the reflectivity, because the electric field on the graphene is zero ( Supplementary Fig. 15 ). Although the resonance behaviour varies with the incidence angle, this device yields reasonably large modulation for broad incidence angles ( Supplementary Figs 16–18 ). Figure 3: Graphene-based switchable radar-absorbing surfaces. ( a ) Schematic representation of the resonant device including the graphene capacitor and metallic surface placed at a distance of quarter-wavelength. ( b , c ) Photographs of the front and the back side of the fabricated device. ( d ) The measured microwave reflection at 10.5 GHz plotted against the bias voltage. The red curve shows the reflection in decibel. ( e ) Real-time reflection from the device during periodic charging and discharging. The device yields around 50 dB reflection suppression ratio. ( f ) Broadband reflection spectrum from the device at various bias voltages. The noise floor is at −80 dB. ( g ) Microwave reflection from the device plotted against the bias voltage and the spacer thickness, which defines the distance between the graphene electrodes and metallic surface. ( h ) Variation of the modulation depth of the resonant device with the spacer thickness. When the graphene is at the antinodes, the modulation is around 100%, whereas at the nodes the modulation is close to zero. ( i ) Broadband reflection spectra from the device for three different spacer thickness. Full size image Next, we would like to discuss some device strategies to cover large area and nonplanar surfaces. As microwave has centimetre scale wavelengths, operating these devices over a large area is essential for realistic applications. For this purpose, we developed pixelated surfaces formed by individually addressable hexagonal-shaped devices ( Fig. 4a–c ). Similar type of multipixel devices has been demonstrated in THz frequencies [43] , [59] , [60] , [61] . The individual device ( Fig. 4d ) consists of a graphene capacitor, a solid spacer (2.5-mm-thick cardboard) and metallic back surface (aluminium foil). The microwave reflection from an individual device is shown in Fig. 4e . At 1.5 V, the reflection decreases substantially with a suppression ratio of 1,000. 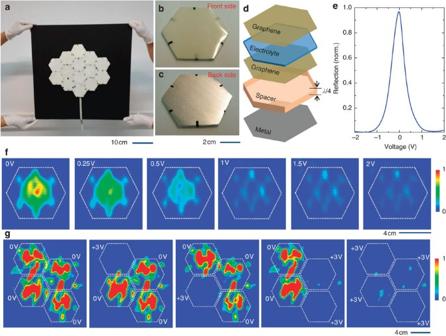Figure 4: Large-area pixelated radar-absorbing surfaces. (a) Photograph of the pixelated microwave surface consists of 14 individually addressable hexagonal-shaped cells. (b,c) Photograph of the front and back side of an individual cell. (d) Exploited view of the structure of an individual cell showing the layers. (e) Microwave reflection of an individual cell at 10.5 GHz. (f) Scanning microwave reflection images of a cell at different bias voltages. (g) Scanning microwave reflection of four cells with different voltage configurations. Figure 4f shows the microwave reflectivity maps of the individual pixel at various voltages. The strong reflection at 0 V diminishes at 1.5 V with slight background reflection due to the contact metals. Then we imaged four cells (scan area is limited by our scanner) at different voltage configurations. When we applied 0 V to the cells we observed reflection from all devices. However, the reflectivity of an individual cell can be suppressed at 3 V. Figure 4g shows reflectivity maps at different voltage configurations. The variation of the reflection within the single cell is due to the reflection from the edges and contact metals. These pixelated surfaces would yield various possibilities for active camouflage systems by shaping the reflectivity pattern from the multipixel adaptive surface. Figure 4: Large-area pixelated radar-absorbing surfaces. ( a ) Photograph of the pixelated microwave surface consists of 14 individually addressable hexagonal-shaped cells. ( b , c ) Photograph of the front and back side of an individual cell. ( d ) Exploited view of the structure of an individual cell showing the layers. ( e ) Microwave reflection of an individual cell at 10.5 GHz. ( f ) Scanning microwave reflection images of a cell at different bias voltages. ( g ) Scanning microwave reflection of four cells with different voltage configurations. Full size image Furthermore, graphene electrodes on flexible polymer substrates allow us to fabricate nonplanar adaptive microwave surfaces as well. 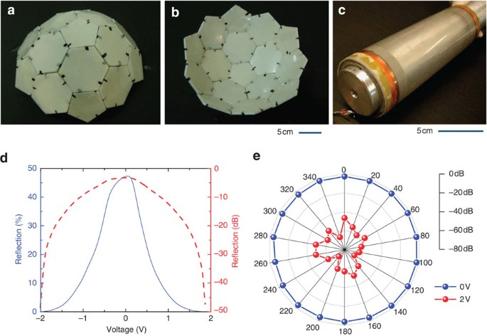Figure 5: Nonplanar adaptive radar-absorbing surfaces. (a,b) Photograph of concave and convex hemispherical surfaces formed by individually addressable hexagon-and pentagon-shaped adaptive cells. (c) Photograph of the cylindrical-shaped switchable radar-absorbing surface placed around a metallic cylinder. The diameter of the cylinder is 4.2 cm. (d) Reflection from the cylindrical surface containing a metallic cylinder as a function of bias voltage. (e) Orientation dependence of the normalized reflection from the surface at 0 and 2 V, respectively. At 2 V the reflectivity is suppressed by 50 dB for all directions. The variation of the intensity on the off-state is due the variation of the distance between the graphene electrodes and metallic cylinder. Figure 5a,b shows concave and convex spherical surfaces formed by multiple individually addressable hexagon- and pentagon-shaped cells. The reflectivity of individual cell (structure shown in the Fig. 4 ) provides reflection suppression of 1,000 for TE polarization. To test an extreme case, we fabricated a cylindrical surface with radius of curvature of 2.6 cm ( Fig. 5c ). Then we placed a metallic cylinder inside the device and measured the reflection from surface at various bias voltages. Figure 5d shows the variation of the microwave reflection from the cylindrical surface as a function of voltage. Even for a large curvature, the microwave reflection is suppressed by 45 dB at 2 V. This modulation is slightly less than the flat resonant surface due to the curvature of the device. The polar plot in Fig. 5e shows the angular dependence of the reflectivity (at 0 and 2 V) of the cylinder obtained by rotating the cylinder around its axis. The polar plot represents tunable radar cross-section of the metallic cylinder. We anticipate that the ability to cover non-planar objects with these active microwave materials will enable new possibilities for microwave cloaking [43] , [47] . Figure 5: Nonplanar adaptive radar-absorbing surfaces. ( a , b ) Photograph of concave and convex hemispherical surfaces formed by individually addressable hexagon-and pentagon-shaped adaptive cells. ( c ) Photograph of the cylindrical-shaped switchable radar-absorbing surface placed around a metallic cylinder. The diameter of the cylinder is 4.2 cm. ( d ) Reflection from the cylindrical surface containing a metallic cylinder as a function of bias voltage. ( e ) Orientation dependence of the normalized reflection from the surface at 0 and 2 V, respectively. At 2 V the reflectivity is suppressed by 50 dB for all directions. The variation of the intensity on the off-state is due the variation of the distance between the graphene electrodes and metallic cylinder. Full size image In summary, we demonstrated a new class of adaptive microwave surfaces using large-area graphene capacitors. We show that graphene electrodes can operate as a tunable Drude metal at microwave frequencies owing to the high-mobility carriers whose density can be tuned by electrostatic doping. Interestingly, this simple device structure yields unprecedented ability to control electromagnetic waves in a very broad spectrum from microwave to the visible spectra. Combining this ability with various device architectures, we demonstrated electrically switchable radar-absorbing surfaces with reflection suppression ratio of 50 dB with operation voltages <5 V. Furthermore, we fabricated various adaptive surfaces including pixelated and nonplanar surfaces. These electrically switchable radar-absorbing surfaces provide technological advantages over the passive microwave absorbers. Our benchmarking studies (see Supplementary Tables 3 and 4 ) show that the key attributes of these adaptive microwave surfaces are the simplicity of device architecture, broadband operation, the mechanical flexibility and potential for low material cost. We believe that these adaptive microwave surfaces will open a new chapter for active camouflage systems, which could find immediate applications in radar technologies. Furthermore, integration of these adaptive surfaces with metamaterial could yield tunable adaptive cloaking in microwave frequencies. Synthesis and transfer printing process of graphene We synthesized large-area graphene by chemical vapour deposition on ultra-smooth copper foils (0.1 μm surface roughness) purchased from Mitsui mining and smelting company (LTD, B1-SBS). We used a quartz chamber with a diameter of 8 cm and rolled the graphene foils on a quartz holder. The growth temperature and duration are 1,035 °C and 30 min, respectively. We heated the samples until 1,035 °C under H 2 flow to reduce the oxide layer of the copper foils. During the growth the partial pressure of CH 4 and H 2 gases were 1.5 and 3 Torr and corresponding rate of flows of 40 and 80 sccm, respectively. After terminating the growth by stopping the flow of methane, we cooled the samples down to room temperature. Then we laminated 70-μm-thick PVC sheets on graphene-coated copper foils. Following the lamination, the copper foils were etched in diluted nitric acid solution and dried overnight to reduce the chemical doping of nitric acid on graphene. Transport measurements We measured capacitance and resistance of the graphene capacitors using HP 4284 A precision LCR meter as a function of bias voltage. We applied an AC signal with amplitude of 100 mV together with variable DC voltage to the device. The serial resistance and capacitance were obtained by using a serial capacitance and resistance (Rs-Cs) model. The voltage bias was applied using a Keithly 2400 Source Measure Unit. Microwave measurements We used a 15-mW microwave transmitter (Gun Diode Microwave Transmitter WA-9314B) operating at 10.5 GHz frequency. The reflected and transmitted power is measured using two microwave receivers (Gun Diode Microwave Receiver) attached to Agilent 34410A 61/2 Digit Multimeter. The microwave reflection spectra were recorded using two broadband standard gain horn antennas (7–12 GHz) attached to a network analyser (0.1–18 GHz Agilent E5063A). How to cite this article: Balci, O. et al. Graphene-enabled electrically switchable radar absorbing surfaces. Nat. Commun. 6:6628 doi: 10.1038/ncomms7628 (2015).